Deep-sea hydrothermal vent animals seek cool fluids in a highly variable thermal environment The thermal characteristics of an organism's environment affect a multitude of parameters, from biochemical to evolutionary processes. Hydrothermal vents on mid-ocean ridges are created when warm hydrothermal fluids are ejected from the seafloor and mixed with cold bottom seawater; many animals thrive along these steep temperature and chemical gradients. Two-dimensional temperature maps at vent sites have demonstrated order of magnitude thermal changes over centimetre distances and at time intervals from minutes to hours. To investigate whether animals adapt to this extreme level of environmental variability, we examined differences in the thermal behaviour of mobile invertebrates from aquatic habitats that vary in thermal regime. Vent animals were highly responsive to heat and preferred much cooler fluids than their upper thermal limits, whereas invertebrates from other aquatic environments risked exposure to warmer temperatures. Avoidance of temperatures well within their tolerated range may allow vent animals to maintain a safety margin against rapid temperature fluctuations and concomitant toxicity of hydrothermal fluids. Environmental temperature is a key parameter governing the distribution of life on Earth. Even slight temperature changes can dramatically affect processes from molecular (for example, enzyme activity [1] ) to organismal scales (for example, predation rates [2] ). In more extreme scenarios, exposure to hot and cold temperatures near an animal's lethal limits can induce metabolic depression and a shift to anaerobic pathways [3] as a result of thermally induced hypoxia [4] . In particular, rapid fluctuations can be very stressful to small aquatic ectotherms because their body temperatures equilibrate quickly with environmental temperatures and physiological compensatory mechanisms are energetically costly [5] . Thus, coping with temperature change and minimizing experienced thermal variability drive the evolution of tolerance limits and behaviours that buffer body temperature change in animals [6] , [7] . Many of the critical leaps in our understanding of how temperature regime shapes the thermal biology of ectotherms have been made by comparing the physiology and behaviours of animals along steep environmental gradients that represent extremes in thermal magnitude and variability over large (for example, latitudinal [8] , [9] and altitudinal gradients [10] ) and small spatial scales (for example, intertidal gradients [5] , [11] ). Hydrothermal vents create one of the most thermally variable habitats in which ectotherms live. Hot, toxic hydrothermal fluids (low oxygen, high sulphide, acidic pH, laden with heavy metals) exit at the seafloor and mix with cold, oxygen-rich bottom seawater to create steep, rapidly fluctuating environmental gradients (±5 °C changes over centimetres and minutes) [12] , [13] , [14] , [15] . Tidal pressure and bottom currents influence turbulent mixing behaviour and venting activity, and drive temperature changes of up to 10 °C at timescales of hours and days [16] , [17] . Previous studies have called attention to the remarkable temperatures tolerated by some vent species [18] , [19] , [20] , [21] and have focussed on characterizing physiological tolerance mechanisms [22] , [23] . For instance, the alvinellid worm ( Paralvinella sulfincola ) from Pacific northeast vents remains a record holder among ectotherms for withstanding 55 °C fluids in aquaria [24] and colonizing surfaces that reach 80 °C [25] . Yet, after three decades of opportunities to study the thermal biology of hydrothermal vent animals, it is unknown whether vent species display distinct behavioural mechanisms to cope with a stochastic thermochemical environment. To establish whether the thermal variability of venting fluids is unique on a global scale, we quantified temporal and spatial temperature variability in hydrothermal vent, shallow-water marine (Antarctic, subtidal and intertidal) and freshwater habitats (alpine, temperate and hot springs) using identical sensors. To test whether vent animals display unique thermal behaviours, we targeted species of Phyla Annelida, Arthropoda and Mollusca from diverse aquatic assemblages for standardized experiments in aquaria. We measured the highest temperature occupied by a species along a horizontal gradient (to estimate the upper preferred temperature [26] ) and the upper lethal thermal limit (temperature at which a prolonged heat coma occurs). Applying a mixed-effects model allowed us to test how much variation in the relationship between the upper selected temperature and lethal limit can be explained by habitat, while accounting for lack of independence because of taxonomic structure. We show that hydrothermal vent fauna seek relatively cooler temperatures than other aquatic fauna, providing the first evidence that vent animals retain a large thermal safety margin, perhaps to cope with extreme temperature fluctuations and the persistent threat of exposure to concentrated hydrothermal fluids. In situ thermal variability Spatial and temporal temperature variability in venting fluids was consistently higher than in other aquatic habitats. A 30-logger array used on a sulphide chimney with P. sulfincola ( Fig. 1a ) quantified >1 °C change cm −1 and multiple degree temporal fluctuations as fluid plumes shift ( Fig. 1b–c , Supplementary Movie 1 ). In comparison, the maximum spatial temperature change at a high rocky intertidal position on a mid-day low tide during early summer was 0.4 °C cm −1 over 24 h ( Fig. 1d ), whereas the mean was <0.1 °C cm −1 . 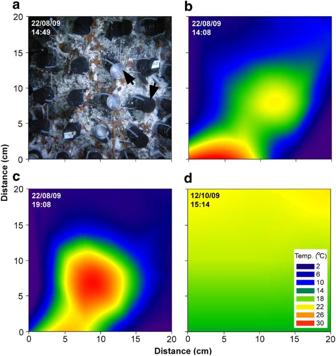Figure 1: Small-scale two-dimensional thermal variability measured with temperature logger arrays. (a) Temperature logger array used at Axial Volcano (1552 m) on a sulphide structure. Twenty-four loggers (two example loggers are indicated by black arrows) are visible among the sulphide worm colony (P. sulfincola). (b,c) Gradients present in venting fluids measured by a logger array at the cm-scale over time. Fluid temperature varies by >1 °C cm−1and fluctuates as fluid plumes shift (Supplementary Movie 1). (d) Maximum gradient present on a rocky intertidal shore (centred at a height of +1.5 m mean low water) in early summer to capture maximum temperature variation between air (25 °C) and surface seawater temperature (15 °C) during the mid-day low tide. Figure 1: Small-scale two-dimensional thermal variability measured with temperature logger arrays. ( a ) Temperature logger array used at Axial Volcano (1552 m) on a sulphide structure. Twenty-four loggers (two example loggers are indicated by black arrows) are visible among the sulphide worm colony ( P. sulfincola ). ( b , c ) Gradients present in venting fluids measured by a logger array at the cm-scale over time. Fluid temperature varies by >1 °C cm −1 and fluctuates as fluid plumes shift ( Supplementary Movie 1 ). ( d ) Maximum gradient present on a rocky intertidal shore (centred at a height of +1.5 m mean low water) in early summer to capture maximum temperature variation between air (25 °C) and surface seawater temperature (15 °C) during the mid-day low tide. Full size image Summary statistics from temperatures recorded at 10-min intervals over 24 h revealed significant differences between vent and non-vent habitats ( n =12 records per habitat category, Supplementary Data 1 ). Although the mean temperature did not differ between vent and non-vent habitats (respectively, 11.51 versus 11.66, multivariate analysis of variance: mean: F 1,22 =0.00, P =0.96), temporal variability was much higher in venting fluids ( Fig. 2 ). Range (10.50 versus 4.37, F 1,22 =11.30, P =0.0028) and standard deviation (2.28 versus 0.95, F 1,22 =7.83, P =0.011) over the 24 h record were twice as high in venting fluids, whereas the absolute value of temperature change between each consecutive 10 min record was at least one order of magnitude greater (0.92 versus 0.065, F 1,22 =54.06, P <0.0001). 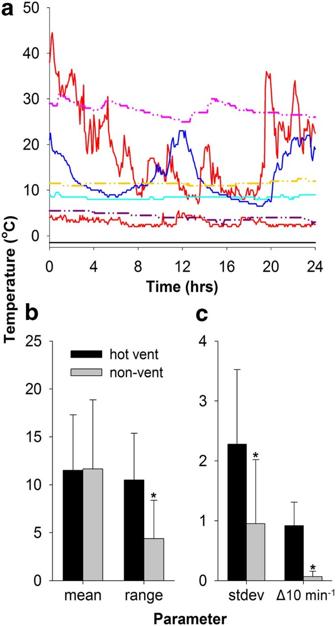Figure 2: Short-term thermal variability in diverse aquatic habitats. Temperatures recorded using identical loggers at 10 min intervals in a variety of aquatic habitats over 24 h. (a) Representative records for marine (solid lines: red, hot vent; blue, intertidal; cyan, subtidal; black, Antarctic) and freshwater (dotted lines: pink, hot spring; orange, temperate spring; purple, alpine run-off) systems over a 24 h period. Hot vent records include a warm and cool habitat (both red solid lines). All other records are from the late spring or early summer seasons (Supplementary Data 1). (b) Temperature mean, range (maximum–minimum), (c) standard deviation and change 10 min−1(absolute difference in temperature between each consecutive 10 min measurement interval) were compared between vent and non-vent aquatic habitats (n=12 pairs,Supplementary Data 1). Whereas mean temperature did not differ by habitat, the three measures of variation were significantly different (indicated by a *, see text for multivariate analysis of variance results). Error bars are +1 s. d. Figure 2: Short-term thermal variability in diverse aquatic habitats. Temperatures recorded using identical loggers at 10 min intervals in a variety of aquatic habitats over 24 h. ( a ) Representative records for marine (solid lines: red, hot vent; blue, intertidal; cyan, subtidal; black, Antarctic) and freshwater (dotted lines: pink, hot spring; orange, temperate spring; purple, alpine run-off) systems over a 24 h period. Hot vent records include a warm and cool habitat (both red solid lines). All other records are from the late spring or early summer seasons ( Supplementary Data 1 ). ( b ) Temperature mean, range (maximum–minimum), ( c ) standard deviation and change 10 min −1 (absolute difference in temperature between each consecutive 10 min measurement interval) were compared between vent and non-vent aquatic habitats ( n =12 pairs, Supplementary Data 1 ). Whereas mean temperature did not differ by habitat, the three measures of variation were significantly different (indicated by a *, see text for multivariate analysis of variance results). Error bars are +1 s. d. Full size image Thermal biology Overall, the upper selected temperature increased with thermal limit ( Fig. 3a , Table 1 , UTL effect: t =11.67, P <0.0001). Although the increase in upper selected temperature with temperature limit was steeper in vent versus non-vent habitats (respectively, 1.10 versus 0.99), the interaction term was not significant ( Table 1 ). However, vent species had significantly lower preferences for any given upper thermal limit than non-vent species, independently of taxonomic affinity ( Fig. 3a , Table 1 , intercept effect (non-vent versus vent): t =3.31, P =0.0037). Much of the taxonomic variation in the upper selected temperature (% variance) occurred at the levels of class, genus and species ( Table 1 ). 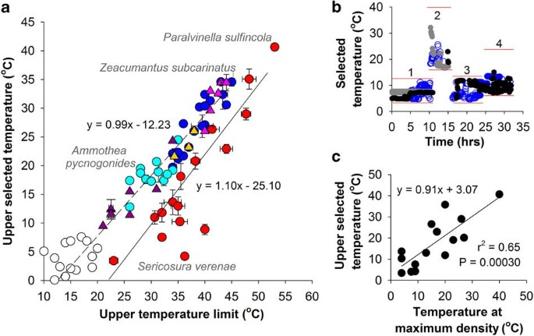Figure 3: Thermal preferences of diverse fauna. (a) Upper thermal limits relate to the upper selected temperatures of 77 species from marine and freshwater habitats that vary in thermal magnitude. Mean (±1 s.e.) is shown for species in which multiple populations were measured. A minimum-adequate linear mixed-effects (LME) model fitted using maximum likelihood included upper selected temperature by upper thermal limit and habitat (marine: red, hot vent; blue, intertidal; cyan, subtidal; black open circles, Antarctic; freshwater: pink, hot spring; orange, temperate spring; purple, alpine run-off), controlling for the random effect of taxonomic non-independence (Table 1). Vent species have significantly lower preferences for any given upper thermal limit than do non-vent species (t=9.77,P<0.0001). Best-fit regression lines for vent (solid) and non-vent habitats (dashed) are based on LME model results. Named species are mentioned in the text of the main article. (b) Temperatures selected by snails (D. globulus, black filled circles), limpets (L. fucensis, grey filled circles) and a scale worm (Branchinotoglumasp., blue open circles) exposed to four different temperature gradients (labelled 1–4) applied in a time series (the upper and lower temperature of each gradient are indicated by red lines). Symbols indicate the temperature selected by each individual every 5 min for the experiment duration. Both limpets remained in the cool end of the chamber after the application of the steep gradient (17–40 °C) and the temperatures occupied by these two limpets were consequently removed from 15 h onwards. (c) The fluid temperature in tubeworm bushes (which are colonized by animals) corresponding to the maximum density of 15 Juan de Fuca Ridge species predicts their upper selected temperatures (determined usingin vitroexperiments).Table 2provides the number of tubeworm bushes collected for each species; as well as the vent fluid temperature and location where maximum animal density occurred. Figure 3: Thermal preferences of diverse fauna. ( a ) Upper thermal limits relate to the upper selected temperatures of 77 species from marine and freshwater habitats that vary in thermal magnitude. Mean (±1 s.e.) is shown for species in which multiple populations were measured. A minimum-adequate linear mixed-effects (LME) model fitted using maximum likelihood included upper selected temperature by upper thermal limit and habitat (marine: red, hot vent; blue, intertidal; cyan, subtidal; black open circles, Antarctic; freshwater: pink, hot spring; orange, temperate spring; purple, alpine run-off), controlling for the random effect of taxonomic non-independence ( Table 1 ). Vent species have significantly lower preferences for any given upper thermal limit than do non-vent species ( t =9.77, P <0.0001). Best-fit regression lines for vent (solid) and non-vent habitats (dashed) are based on LME model results. Named species are mentioned in the text of the main article. ( b ) Temperatures selected by snails ( D. globulus , black filled circles), limpets ( L. fucensis , grey filled circles) and a scale worm ( Branchinotogluma sp., blue open circles) exposed to four different temperature gradients (labelled 1–4) applied in a time series (the upper and lower temperature of each gradient are indicated by red lines). Symbols indicate the temperature selected by each individual every 5 min for the experiment duration. Both limpets remained in the cool end of the chamber after the application of the steep gradient (17–40 °C) and the temperatures occupied by these two limpets were consequently removed from 15 h onwards. ( c ) The fluid temperature in tubeworm bushes (which are colonized by animals) corresponding to the maximum density of 15 Juan de Fuca Ridge species predicts their upper selected temperatures (determined using in vitro experiments). Table 2 provides the number of tubeworm bushes collected for each species; as well as the vent fluid temperature and location where maximum animal density occurred. Full size image Table 1 Summary of mixed-effects model results. Full size table After a 1-week recovery at habitat pressure, individuals of three hydrothermal vent species displayed preferences for low temperatures in a 30 h-long experiment, in which four temperature gradients that varied in magnitude were applied in series ( Fig. 3b ). Whereas animals moved throughout the chamber when the gradient ranged from 4 to 10 °C, on application of a steeper but realistic gradient (17–40 °C), the scale worm ( Branchinotogluma sp.) selected the coolest corner of the aquarium, followed by snails ( Depressigyra globulus ) and limpets ( Lepetodrilus fucensis ). When temperature was decreased (4–12 °C), limpets remained in the cool end of the aquarium and did not move during the latter half of the experiment, whereas the worm and snails were active throughout the aquarium. When a steeper temperature gradient was again established (7–24 °C), the worm and snails consistently selected temperatures <15 °C. There was direct correspondence between the habitat temperatures occupied by 15 Juan de Fuca Ridge vent species and their respective upper selected temperature in experimental aquaria. Specifically, the maximum fluid temperature measured in a tubeworm bush in which the highest density of a species was observed ( Table 2 provides sampling details) related to its upper selected temperature: the slope of this relationship for the 15 species was near one (0.91) and the intercept approached zero (3.01) ( Fig. 3c ). Table 2 Vent species included in a comparison of in situ and in vitro temperature preferences. Full size table We propose that vent fauna maintain a wider thermal safety margin than other aquatic invertebrates in response to the extreme spatial and temporal environmental variability presented by vent fluids ( Supplementary Movie 1 ). Temperature records in all aquatic habitats sampled using identical loggers provide the first standardized measurements directly comparing short-term temporal temperature variability among diverse habitats at scales relevant to the body temperature of small animals. Diffuse vent habitats are characterized by order of magnitude higher spatial and temporal temperature variability. Even in high intertidal habitats, which are a model system for studies of thermal variability and in which we measured a single-day temperature change from 5.0 to 26.5 °C ( Supplementary Data 1 ), the variation followed a predictable pattern (sinusoidal function reflecting tidal pattern), allowing for short-term (many hours) temperature responses [5] . In addition to being unique in seeking relatively cool temperatures compared with their heat tolerance, mobile vent species displayed conspicuous escape responses, such as thrashing, and marked increases in movement when exposed to temperatures approaching their upper thermal limit. Such behaviours may increase their chances of finding a cooler environment. Indeed, behavioural avoidance is a primary defence used by ectotherms from the tropics and deserts to prevent exposure to dangerously hot temperatures [27] . Thus, for sessile vent species, microhabitat selection may be even more important to avoid environmental fluctuations that broach physiological thresholds. In comparison, animals from other aquatic habitats selected fluids that exceeded their expected long-term acute limits, even when experiments were extended to 24 h in duration. For instance, an intertidal snail ( Zeacumantus subcarinatus : Fig. 3 ) retracted into its shell after 12 h at 35 °C instead of moving to cooler areas of the chamber. In experiments conducted with Antarctic species, well known for adaptation to a highly stenothermal environment [28] , a few individuals in each trial would move into fluids with temperatures (>7 °C) that initiated a coma, and all but two species ( Harmathoe sp. and Nymphon sp.) displayed no escape responses during the determination of upper thermal limits. Even vent species that selected cool fluids (2–5 °C) displayed thermal limits that were >30 °C. Most striking is the difference between thermal limits and preferences of two related pycnogonid sea spiders (family Ammotheidae) from a vent and subtidal habitat (respectively, Sericosura verenae and Ammothea pycnogonides ). The vent pycnogonid withstood temperatures of up to 36 °C in spite of actively avoiding fluids >5 °C, whereas the subtidal species was less tolerant to heat (upper limit=31 °C) but selected fluids up to 20 °C. Finding that peripheral vent fauna in fluids <5 °C can survive exposure to high temperatures is surprising because cold adaption is generally thought to relate to reduced heat tolerance [4] . Longer-term thermal preference experiments and in situ temperature distribution patterns strongly support the fact that it is unlikely that our results are due to decompression stress upon collection of hydrothermal vent animals. Individuals of three vent species provided with a 1-week recovery at their habitat pressure, followed by exposure to a series of thermal gradients, consistently selected the coolest area of the gradient aquarium ( Fig. 3b ). Moreover, the direct correspondence between natural patterns and laboratory experiments provides unequivocal evidence that Juan de Fuca vent species prefer habitats with moderate temperatures <20 °C [14] . Although factors such as food availability [19] likely also influence the thermal preferences of vent fauna, our results point to understanding how vent animals persist in a highly stochastic habitat as a key direction for future research. Even in cool microhabitats in which animals are abundant, the degree of temperature variability sustained by individuals on a minute-to-minute basis is extreme. Thus, sublethal effects at moderate temperatures may also be important. For example, a deep-sea vent shrimp ( Rimicaris exoculata ) produces an inducible heat-shock protein (in the hsp70 family) at <25 °C [29] . A recent study has also shown that increasing temperature above 25 °C induces metabolic depression in a vent mussel ( Bathymodiolus azoricus ) [30] . These coping mechanisms are energetically costly and highlight the potential importance of behavioural avoidance in preventing exposure to high temperatures in the first place. The occurrence of high temperatures that correspond to low oxygen, high sulphide, acidic pH and high metal concentrations, combined with extreme spatial and temporal variability, is unique to hydrothermal habitats. Here, we show that temperature is an important environmental signal for the fauna of vents that may minimize exposure to a combination of potentially deleterious environmental stresses [14] . Rather than temperature alone, the associated toxic chemical milieu and inherent variability of vent habitats that accompanies increasing vent fluid temperatures may drive the evolution of low thermal preferences that reduce the likelihood of death. Behavioural mechanisms such as 'playing it safe' may be equally as important as physiological tolerance in allowing animals to thrive in variable environmental conditions. In situ temperature. Temperature loggers were DS1921 Thermochron ibuttons (±0.5 °C) enclosed in titanium housings with polycarbonate endcaps [31] ( Fig. 1a ). Spatial patterns in temperature were derived from logger arrays set to record temperature every 2 min in active vent flow with abundant animals (5×6 grid, spaced 5 cm apart [4 loggers failed during the deployment]) and at a high intertidal location during summer (3×3 grid, spaced 10 cm apart). Identical single loggers were also used in various habitats to capture temporal patterns by logging temperature at 10 min intervals. Summary statistics for each location were quantified from a 24 h record. See Supplementary Data 1 for further details. Thermal biology. We conducted standardized experiments using identical aquaria to quantify the upper selected temperature and the upper lethal limit at 20 (Endeavour and Middle Valley fauna) or 15 MPa (Axial fauna) or surface pressure (non-vent fauna) with fluid inflow at 1 ml min −1 . Aquaria were designed with clear polycarbonate windows to allow the determination of individual position and viewing under a light microscope ( Fig. 4 ). Supplementary Data 2 summarizes specimen collection details, taxonomy, body length, sample sizes and experimental fluid temperatures. Replicate trials for the same species were conducted, where feasible, with animals from different locations or seasons to capture variability in thermal biology due to thermal history. 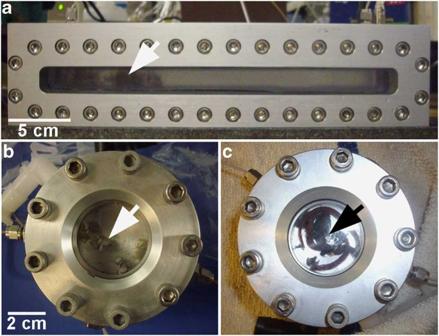Figure 4: Experimental aquaria. Vent animals (indicated by arrows) visible through polycarbonate windows in the (a) thermal gradient aquarium and (b,c) thermal limit aquaria. Figure 4: Experimental aquaria. Vent animals (indicated by arrows) visible through polycarbonate windows in the ( a ) thermal gradient aquarium and ( b , c ) thermal limit aquaria. Full size image We tested for habitat-related differences in upper selected temperature versus thermal limit using a hierarchical linear mixed-effects model, with body length as a fixed factor and taxonomic structure (nested as phylum, class, family, genus, species) as a random effect on the intercept ( nLME package, R 2.8.1: R Development Core Team, 2009) [32] . To compare the thermal response of animals from the same range of habitat temperatures experienced at deep-sea hydrothermal vents, we first tested for significant differences in the intercept of the relationship between upper selected temperature and upper thermal limit among the three shallow marine (intertidal, subtidal and Antarctic) and also among three freshwater categories (hot spring, temperate spring and alpine run-off) with analysis of covariance, using the mean values for species, except in cases in which only one population was measured; the intercept did not differ among the subhabitat categories in either case (analysis of covariance results: marine, F 2,41 =0.90, P =0.41; and freshwater, F 2,12 =1.22, P =0.33). Thus, we began with a mixed-effects model that included three habitats (categorical variables: vent, shallow marine and freshwater) with continuous representation across a similar range in upper temperature limits and body length (numeric variable: size). The full model included all higher-order interactions, followed by identification of the minimum adequate model by stepwise removal of non-significant terms [32] . Body length (size) was removed as a fixed factor because its effect on the reference intercept and slope was not significant. Marine and freshwater habitats were collapsed into one category (non-vent) during model simplification. Upper selected temperature. To estimate the upper preferred temperature [26] , we measured the highest temperature selected by a species along a horizontal temperature gradient (Antarctic specimens: −1.8 to 15 °C, P. sulfincola : 10–50 °C, all other fauna: 2–40 °C). The gradient was maintained by cooling one end of an aluminium aquarium with a re-circulating water bath and heating the opposite end with an electric heating element [9] . Animals had unrestricted access along a slot 33 cm long×1.0 cm wide×1.5 cm high) in the gradient aquarium that was fitted with a strip of mesh (0.5 mm Nitex, to provide a rough surface). Before applying the temperature gradient, we ensured that animals occupied a uniform distribution (except in the Antarctic species, in which we jostled animals to the cold end because 12 of the 14 species did not respond to high temperature with escape responses). Black plastic was draped over the chamber during trials with all non-vent animals to exclude light as a selection cue. We measured the temperature gradient with a digital thermometer probe (VWR, ±0.2 °C) placed in 3.18 mm holes spaced at intervals of 1 cm along the length of the aquarium. The temperature corresponding to the position of each individual was recorded after 3 h; upper selected temperature was used as the relevant parameter because avoidance behaviour was of interest. Each trial consisted of 5–30 individuals per species depending on availability and body length ( Supplementary Data 2 ). Vent animals were collected from a depth of ∼ 2200 m (Endeavour and Middle Valley) and placed immediately in pressurized aquaria (20 MPa) for 3 h before the start of experiments. To confirm that decompression does not significantly alter thermal preferences, we conducted gradient experiments with three species (limpet: L. fucensis ; snail: D. globulus ; and scale worm: Branchinotogluma sp.) collected at 1500 m depth (Axial Volcano, ASHES vent field) and held at pressure for 1 week ( ∼ 10 °C) to allow recovery. Different temperature gradients that varied in magnitude were then applied in series to these specimens from Axial while the position of each individual was recorded at 5 min intervals over 3 days. To determine whether longer experimental durations result in lower selected temperatures, we held four non-vent species in the gradient aquaria for 24 h: Paramoera walkeri (Antarctic), Potamophyrgus antipodarum (temperate spring), Physa acuta (hot spring) and Z. subcarinatus (intertidal) (20 individuals of each species). We did not detect significant differences in temperature distributions between the 3- and 24-h gradient experiments in these four species (the Kolmogorov–Smirnov test). Upper lethal thermal limit. Animals ( Supplementary Data 2 ) were heated in one degree increments (each heating cycle lasted 15 min), spaced by a recovery stage at a cool temperature (15 min) to allow for comparison among fauna with different behaviours on heating: for example, snails retract at sublethal temperatures but respond on return to cooler fluids. The temperature at which all individuals remained unresponsive during observation under a light microscope (=coma) was recorded as the upper lethal thermal limit. Internal aquarium fluid temperature (internal chamber dimensions: height=76 mm, diameter=30 mm) was controlled by submerging the aquarium in a water bath and monitored with a digital thermometer (VWR, ±0.2 °C) with the probe tip fitted to contact the chamber fluid. In situ density and thermal niche. Vent tubeworm ( Ridgeia piscesae ) bushes ( n =33; Table 2 ) were collected by submersible (Pisces IV, Alvin or ROPOS) at vents along the Juan de Fuca Ridge and fixed in formalin. Animals were counted and, for each species present, density was standardized to the surface area of R. piscesae tubes [33] . Maximum habitat temperature was measured by holding a single temperature probe in venting fluids for ∼ 10 min. How to cite this article: Bates, A.E et al . Deep-sea hydrothermal vent animals seek cool fluids in a highly variable thermal environment. Nat. Commun. 1:14 doi: 10.1038/ncomms1014 (2010).